Adding control to arbitrary unknown quantum operations Although quantum computers promise significant advantages, the complexity of quantum algorithms remains a major technological obstacle. We have developed and demonstrated an architecture-independent technique that simplifies adding control qubits to arbitrary quantum operations—a requirement in many quantum algorithms, simulations and metrology. The technique, which is independent of how the operation is done, does not require knowledge of what the operation is, and largely separates the problems of how to implement a quantum operation in the laboratory and how to add a control. Here, we demonstrate an entanglement-based version in a photonic system, realizing a range of different two-qubit gates with high fidelity. Perhaps the most notable future application of quantum science is quantum information processing, which promises secure communication [1] and greatly increased speeds for solving certain problems such as database searching [2] , factoring [3] and quantum simulation [4] . The excitement surrounding quantum computers lies in the fact that the number of elementary operations that they require to solve these problems scales only polynomially with the size of the input, in contrast to exponential scaling on a conventional computer. However, even a polynomial scaling of quantum computational resources still presents an enormous obstacle to practical realization. It may well be that although a quantum computer could, in principle, efficiently solve these important problems, it will remain practically infeasible to build one that can implement a sufficient number of operations, on enough qubits and with sufficient precision, to do anything useful. This motivates developing methods to reduce the resource overhead required to implement key quantum algorithms. Quantum algorithms rely on the decomposition of a functional quantum circuit into an elementary logic gate set, such as that formed by single-qubit and two-qubit controlled-NOT (CNOT) gates [5] ; there have been several experiments to demonstrate universal quantum gate sets in different physical architectures [6] including ion traps [7] , [8] , linear optics [9] , [10] , [11] , [12] , [13] , superconductor [14] , [15] , atoms [16] , [17] , and even small-scale algorithms [18] , [19] , [20] , [21] . However, the large number of elementary gates required to implement even the modest-sized circuits presents a significant challenge. This complexity is due to not only the sheer number of elementary operations required but also the structure in which these gates are combined. Controlled-unitary (CU) gates are a particularly important class of circuits, where one 'control' qubit turns on or off a unitary operation U acting on a register of 'target' qubits ( Fig. 1a ). These circuits feature heavily in Kitaev's phase estimation algorithm [22] that underpins Shor′s factoring algorithm [3] and quantum simulation [4] . In the context of quantum simulation, U could represent a simulation of the time-evolution operator of some physical system, and the ability to add control qubits allows energy eigenvalues to be read out through the phase estimation algorithm [23] . Phase estimation is also a fundamental tool in quantum metrology. However, the current standard method of realizing CU gates, which relies on the decomposition of U into an elementary gate set, may not be suitable for these applications: in Kitaev's phase estimation algorithm U may be an unknown 'black box' that cannot be decomposed at all. 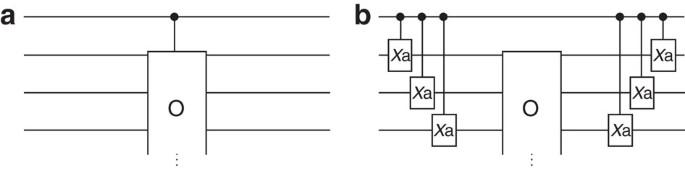Figure 1: Controlling arbitrary quantum operations using additional degrees of freedom. (a) Logic circuit in which quantum operation O is implemented on a register of qubits (target register), conditional on the logical state of a single control qubit. (b) Our approach to implementing the circuit in (a). The target information carriers are four dimensional systems with logical states |0〉,|1〉,|2〉 and |3〉. Initially and finally, only the bottom two 'qubit' levels (|0〉 and |1〉) are populated. Controlled-Xagates (equations 1 and 2) swap information between the qubit levels and the upper levels (|2〉 and |3〉), on which O does not act. In this way, conditional on the state of the control qubit, the entire quantum state of the target register is temporarily moved into an effective quantum memory on which O does not act. Figure 1: Controlling arbitrary quantum operations using additional degrees of freedom. ( a ) Logic circuit in which quantum operation O is implemented on a register of qubits (target register), conditional on the logical state of a single control qubit. ( b ) Our approach to implementing the circuit in ( a ). The target information carriers are four dimensional systems with logical states |0〉,|1〉,|2〉 and |3〉. Initially and finally, only the bottom two 'qubit' levels (|0〉 and |1〉) are populated. Controlled- X a gates (equations 1 and 2) swap information between the qubit levels and the upper levels (|2〉 and |3〉), on which O does not act. In this way, conditional on the state of the control qubit, the entire quantum state of the target register is temporarily moved into an effective quantum memory on which O does not act. Full size image Here we present and demonstrate a simple method for realizing controlled quantum operations (CO), of which CU gates are a subset. In the following we first explain the technique in a way that is independent of any particular physical system, before describing a conceptual example in a photonic system. We then show that the equivalent operation can be achieved by exploiting an entangled initial state—reminiscent, but distinct from, cluster state quantum computing [24] , [25] . Finally, we apply this approach in a series of proof-of-principle experiments implementing various two-qubit gates which include a CNOT, a number of other CU gates, as well as 'entanglement-filter' and 'entanglement-splitter' gates. Explanation of the general technique Our approach for adding a control qubit to an arbitrary quantum operation O is shown conceptually in Figure 1b . In summary, conditional on the logical state of the control, the quantum state of the target register ( ψ ) is temporarily shifted into a part of an extended Hilbert space on which O does not act (imparts the identity operation). In this way the evolution of ψ is dependent on the control qubit state, if it is |0〉 (|1〉) then ψ→ψ (ψ→Oψ ). The Hilbert space is extended by employing an extra two levels in each quantum information carrier in the target register, making each a four-level system with logical states |0〉,|1〉,|2〉 and |3〉. The action of each X a gate is to swap information between the bottom two 'qubit' levels (|0〉, |1〉) and the expanded Hilbert space (|2〉, |3〉), that is, In spite of its conceptual simplicity, the technique has significant practical benefits: it largely separates the experimental problems of how to implement any given quantum operation in the laboratory and how to add a control qubit. This is relevant in many experimental cases where it is not at all clear how to directly add a control to a quantum operation, for example, when O can be realized in analogue fashion by turning on an experimental hamiltonian, or when O is a non-unitary operation implemented by directly coupling to a bath. Even in the case where O can be constructed with a universal gate set, the number of additional operations required to add a control will generally be far less following our approach. Furthermore, in situations where O is unknown, our method may be the only way to add control. This is relevant in quantum metrology where the goal is to measure properties of O. The method can be straightforwardly extended to realize the conditional implementation of two different operations O 1 or O 2 based on the state of the control qubit. Here whereas the component of the state that is unmoved undergoes O 1 , the component of the state moved into the expanded Hilbert space undergoes O 2 . A further extension would be to add multiple control qubits to implement one of several quantum operations, based on the state of all of the control qubits. For example, with two control qubits, four operations O 1 , O 2 , O 3 , or O 4 could be implemented depending on the state of the control qubits. An alternative approach to extending the Hilbert space would be to use another register of qubits and controlled-swap operations to move information between the registers. However, whereas adding more qubits has proved to be a significant experimental challenge, multi-dimensional quantum information carriers are readily available in most physical systems currently being investigated or used for quantum information processing. Trapped ions systems, for example, offer a large number of precisely controllable internal electronic and external vibrational degrees of freedom. Our technique could be implemented by conditionally moving quantum information between different electronic transitions, on which subsequent operations do not operate, or operate differently, on. We note that in previous work it was shown how moving part of the state of a target qubit into an expanded Hilbert space can simplify adding control qubits [26] . However, this only works in the case where the target is a single-qubit unitary and is at the expense of changing how the unitary must be implemented. Optical version of the scheme Although our technique is independent of the particular physical system and degree of freedom employed, it is particularly well suited to an optical version in terms of the polarization and spatial degrees of freedom of photonic qubits. 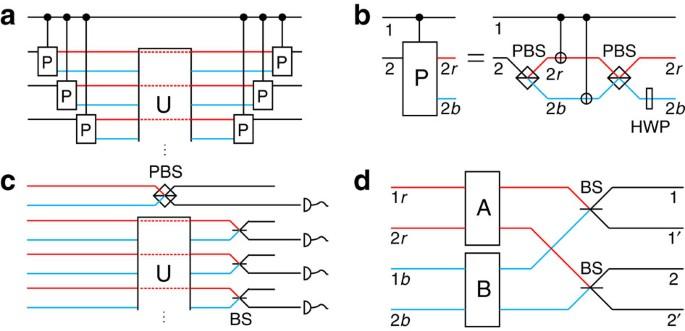Figure 2: Optical implementation of the scheme. (a) Implementation of a CU gate. The circuit is composed of three parts: controlled-path gates (CP) at the beginning, which move the target qubits from upper spatial modes (labelled red) to lower spatial modes (labelled blue) if the control qubit is in the logical state |1〉; the unitary gate U in the middle is implemented on the lower spatial modes; and CPs at the end, which combine the upper and lower spatial modes. (b) Construction of a CP gate. When the control is in the logical state |0〉, nothing is applied on the target and the photon exits in the red mode. When the control is |1〉, the polarization of the target flips and the photon exits in the blue mode. HWP flips back the polarization of the target photon in the blue mode. (c) Entanglement-based scheme. Instead of implementing CPs before the unitary gate U, one sets the input state in an equal superposition of photons either all in the red modes or all in the blue modes. The CPs after U are substituted by a series of non-polarization BS. (d) Linear combinations of quantum operations . The two photons are either in the red modes 1r,2ror in the blue modes 1b,2bwhich pass through quantum operations A and B, respectively. Then two spatial modes 1r,1b(2r,2b) of photon 1 (2) are combined at a BS. By postselecting two photons at ports 1,2 or 1′,2′ (1,2′ or 1′,2), one can effectively realize the quantum operationA+B(A−B). As shown in Figure 2a , the controlled-path (CP) gate substitutes the C X a in Figure 1b . The CP is a two-photon gate that changes the target photon's path if the control is vertically polarized. We note that the CP gate has previously been proposed for implementing controlled gates in the context of weak optical cross-Kerr nonlinearities [27] , [28] . Figure 2: Optical implementation of the scheme. ( a ) Implementation of a CU gate. The circuit is composed of three parts: controlled-path gates (CP) at the beginning, which move the target qubits from upper spatial modes (labelled red) to lower spatial modes (labelled blue) if the control qubit is in the logical state |1〉; the unitary gate U in the middle is implemented on the lower spatial modes; and CPs at the end, which combine the upper and lower spatial modes. ( b ) Construction of a CP gate. When the control is in the logical state |0〉, nothing is applied on the target and the photon exits in the red mode. When the control is |1〉, the polarization of the target flips and the photon exits in the blue mode. HWP flips back the polarization of the target photon in the blue mode. ( c ) Entanglement-based scheme. Instead of implementing CPs before the unitary gate U, one sets the input state in an equal superposition of photons either all in the red modes or all in the blue modes. The CPs after U are substituted by a series of non-polarization BS. ( d ) Linear combinations of quantum operations . The two photons are either in the red modes 1 r ,2 r or in the blue modes 1 b ,2 b which pass through quantum operations A and B, respectively. Then two spatial modes 1 r ,1 b (2 r ,2 b ) of photon 1 (2) are combined at a BS. By postselecting two photons at ports 1,2 or 1′,2′ (1,2′ or 1′,2), one can effectively realize the quantum operation A+B ( A−B ). Full size image To understand how the CP gate works, let's examine its structure shown in Figure 2b . Assume the inputs are two polarization-encoded photonic qubits, α | H 〉 1 + β | V 〉 1 (control photon 1) and γ | H 〉 2 + δ | V 〉 2 (target photon 2). The first polarizing beamsplitter (PBS) will convert the target state from γ | H 〉 2 + δ | V 〉 2 to γ | H 〉 2b + δ | V 〉 2r where 2 r and 2 b denote the red and blue spatial modes of the target photon, respectively. The subsequent two CNOT gates flip the polarization of the target photon, if the first photon is vertically polarized. (It is assumed that if a CNOT acts on an unoccupied spatial mode, the identity is enacted.) Thus, the two-photon state becomes α | H 〉 1 ( γ | H 〉 2 b + δ | V 〉 2 r )+ β | V 〉 1 ( γ | V 〉 2 b + δ | H 〉 2 r ). Then the two spatial modes 2 r and 2 b of the target photon are mixed on the second PBS which converts the two-photon state to α | H 〉 1 ( γ | H 〉 2 r + δ | V 〉 2 r )+ β | V 〉 1 ( γ | V 〉 2 b + δ | H 〉 2 b ). Finally, a half-waveplate (HWP) flips the polarization in spatial mode 2 b and thus converts the state to α | H 〉 1 ( γ | H 〉 2r + δ | V 〉 2r )+ β | V 〉 1 ( γ | H 〉 2b + δ | V 〉 2b ): the result is that the target polarization qubit is to be found in one of two orthogonal spatial modes, depending on the logical state of the control qubit. By defining | H 〉 2b , | V 〉 2b , | H 〉 2r and | V 〉 2r as |0〉, |1〉, |2〉 and |3〉, respectively, one can easily find that a CP exactly realizes the function of a C X a gate. Returning to Figure 2a , suppose that the control photon is again initially in the arbitrary polarization-qubit state α | H 〉+ β | V 〉 and the target photons are initially in the multi-qubit state | ψψ 〉. The photons pass through a sequence of CPs which changes the path of all target photons if the control photon is vertically polarized, thus the state is converted to α | H 〉| ψ 〉 r + β | V 〉| ψ 〉 b where r and b denote the collective red and blue spatial modes, respectively. Next, the blue spatial modes b of the target photons are acted upon by U , whereas the red spatial modes r do not pass through the unitary, as indicated by the dotted lines. The state is therefore converted to α | H 〉| ψ 〉 r + β | V 〉 U | ψ 〉 b . Finally, by repeating the sequence of CPs, we obtain the desired state α | H 〉| ψ 〉+ β | V 〉 U | ψ 〉 at the output. There is a clear advantage over the conventional quantum computational approach to adding control qubits, in terms of the number of logic gates required. Assuming that U, which is a unitary acting on n qubits, can be decomposed into a circuit of p CNOTs and q single-qubit gates, one would use p Toffoli gates and q two-qubit controlled gates to build the corresponding CU gate, which can further be decomposed into (3 p+q ) to (6 p+ 2 q ) CNOTs and even more single-qubit gates [29] . Although 4 n more CNOTs suffice to add a control to the n-qubit unitary U by using our method, at least (2 p+q ) more CNOTs are needed if one sticks to the traditional scheme. For most quantum algorithm applications, such as Shor′s algorithm where U is a modular exponentiation gate, the typical value of ( p+q ) is about 72 n 3 which is on the order of O( n 3 ) and thus (2 p+q ) is much larger than 4 n when n becomes large [29] , [30] . Furthermore, if U is a non-unitary operation, then the conventional approach is to rewrite this as a unitary on a larger Hilbert space, at a significant cost to the number of gates required. There is no additional cost to add controls to non-unitary operations following our approach. Entanglement-based scheme Even a two-qubit demonstration of our scheme would require two CP gates and subsequently four CNOT gates, which is presently out of reach using current linear-optical quantum information processing technology. However, the effect of the CP gate is to generate entanglement between the control qubit and target register, and this kind of entanglement can be generated directly from existing photon sources. We now present an alternative entanglement-based version of our scheme which is feasible with current technology. Consider the optical circuit schematic shown in Figure 2c . At the input, a spatially-entangled n -photon state is injected that is an equal superposition of finding one photon in each of the n red modes and one photon in each of the n blue modes. In the case where the polarization of the n -photon input state is | φ 〉=( α | H 〉+ β | V 〉)| ψ 〉, where α | H 〉+ β | V 〉 is the upper control qubit and | ψ 〉 is the joint state of the lower ( n –1) target register qubits, then the initial state can be written as where r and b label the collective red and blue spatial modes, respectively, and | vac 〉 represents an unoccupied mode. From now on we will drop the unoccupied vacuum modes from the notation. Note that, as we will show, it is possible to create such a state from a spontaneous parametric down conversion photon source. The quantum operation U acts only on photons in the blue spatial modes of the target register. The information about whether the target state ψ does or does not undergo the operation U is therefore encoded in the spatial mode of the control photon. Mixing the two control modes on a PBS and postselecting on finding the control photon in the lower spatial mode move this information into the polarization of the control photon, yielding the state: Finally, the red and blue modes of each target qubit are mixed on non-polarising beamsplitters (BS) to remove the path information. In the case where all photons exit in the lower paths, the output state is as required. The probability of success is (1/2) n , however all combinations of the control photon arriving in lower spatial mode and an even number of target photons arriving in lower spatial modes will give a state with the same form as in equation 5. There are 2 n –2 such combinations that the total probability of success is 1/4, regardless of the number of qubits U acts on. The important feature of our approach —that any operation (known or unknown) can be controlled without changing the way the operation is done—is retained in the entanglement-based approach. This approach can be reformulated in a more general way as shown in Figure 2d . Here we consider the two-photon case for simplicity. Beginning with the two-photon input state of equation 3, the red and blue modes pass through quantum operations A and B respectively. The state is obtained. After mixing the spatial modes on the two BSs, one would get ( A+B )| φ 〉 if the two photons exit at ports 1 and 2 or 1′ and 2′. Otherwise, if the two photons exit at ports 1 and 2′ or 1′ and 2, ( A–B )| φ 〉 would be obtained. To realize the CU gate, one just needs to set A= | H 〉〈 H | I and B= | V 〉〈 V | U , where | H 〉〈 H | and | V 〉〈 V | denote projectors onto | H 〉 and | V 〉, respectively. This approach provides a new perspective on constructing quantum gates: Whereas the traditional decomposition method can be regarded as performing multiplication, which corresponds to rewriting the target gate matrix as the product of several gate matrices, our method is performing linear combination, which means rewriting the target gate matrix as the sum of several gate matrices. This entanglement-based scheme would be useful for small-scale applications as well as subroutines in larger calculations, and it could be made deterministic, following the original prescription for linear optical quantum computation [31] . Introducing nonlinearities is another way to approach a unit success probability [27] . Experimental demonstration We now present experimental demonstrations of several two-qubit CU gates using this general entanglement-based method (specifically corresponds to Fig. 2d ). 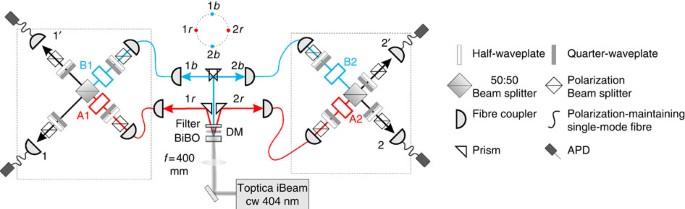Figure 3: Experimental setup for realizing CU gates. A 60 mW continuous-wave (CW) laser beam with a central wavelength of 404 nm is focused onto a BiBO crystal to create photon pairs. Both the horizontal (modes 1rand 2r) and vertical (modes 1band 2b) photon pairs are collected. Before collection into polarization-maintaining fibres (PMF), the photons are spectrally filtered by narrow-band filters (ΔλFWHW=3.2 nm). A1, B1, A2 and B2 are four single-qubit gates. By post-selecting the case the two photons exit at ports 1 and 2, one would effectively realize a two-qubit quantum gate (A1A2+B1B2). The phase between the two components is stabilized by monitoring the coincidence count rates between detectors 1′ and 2′. Figure 3 shows a schematic diagram of our experiment. Note the simplicity of this scheme relative to the previous demonstration of photonic CU gates [26] , in particular, the fact that it requires no quantum interference. A continuous-wave laser is focused onto a BiBO crystal and thus produces photon pairs through the type-I spontaneous parametric-down conversion (SPDC) process. We collect two photons from four points from the SPDC cone, as shown, resulting in a two-photon four-mode state [32] of the form . By passing each mode through several waveplates, we prepare a state , where | φ 〉 can be an arbitrary two-qubit separable state. Here we designate photon 1 as the control, which is in modes 1 r and 1 b , and photon 2 as the target, which is in modes 2 r and 2 b . Before modes 1 r (2 r ) and 1 b (2 b ) are combined at a BS, we let the four modes pass through four single-qubit gates A 1, B 1, A 2 and B 2 that are constructed from waveplates or PBSs. Then, by measuring the two-photon coincidences between detectors at ports 1 and 2, we get the state ( A+B )| φ 〉, where A=A1 A 2 and B=B1 B 2. As explained above , by setting A 1=| H 〉〈 H |, A 2= I , B 1=| V 〉〈 V | and B 2= U , the corresponding CU gate is obtained. Figure 3: Experimental setup for realizing CU gates. A 60 mW continuous-wave (CW) laser beam with a central wavelength of 404 nm is focused onto a BiBO crystal to create photon pairs. Both the horizontal (modes 1 r and 2 r ) and vertical (modes 1 b and 2 b ) photon pairs are collected. Before collection into polarization-maintaining fibres (PMF), the photons are spectrally filtered by narrow-band filters (Δ λ FWHW =3.2 nm). A1, B1, A2 and B2 are four single-qubit gates. By post-selecting the case the two photons exit at ports 1 and 2, one would effectively realize a two-qubit quantum gate (A1 A2+B1 B2). The phase between the two components is stabilized by monitoring the coincidence count rates between detectors 1′ and 2′. Full size image We constructed a series of CU gates, including CNOT, C-Hadamard (CH), CPhase (CZ), CZ( π /2) and CZ( π /4) gate, by setting B 2 =X,H,Z,Z π/2 〈 and Z π/4 , respectively. To evaluate the performance of these gates, we adopted the method introduced in ref. 33 . For each gate, two truth tables are measured in complimentary bases. 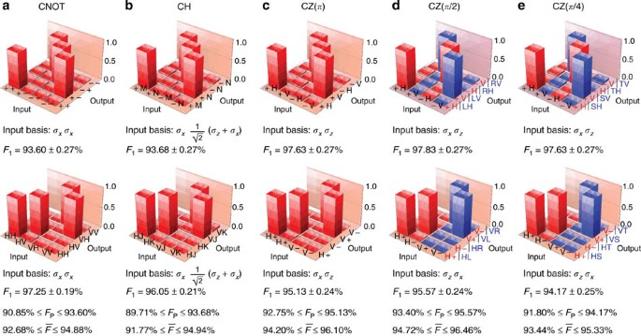Figure 4: Implementing two-qubit controlled-unitary operations by harnessing entanglement in a larger Hilbert space. (a–e) Experimentally measured 'truth tables' for several CU gates. For the inputs of the CH gate |M〉 and |N〉 (|J〉 and |K〉) are the eigenstates ofwith +1 and −1 eigenvalues respectively: that is |M〉=cos(π/8)|H〉+sin(π/8)|V〉; |N〉=sin(π/8)|H〉−cos(π/8)|V〉; |J〉=cos(5π/8)|H〉+sin(5π/8)|V〉; |K〉=sin(5π/8)|H〉−cos(5π/8)|V〉. Note that two different output measurement bases are applied for each truth table of CPhase(π/2) and CPhase(π/4). The red columns correspond to red output labels whereas the blue columns correspond to blue output labels, which include states such as |HL〉, |HR〉, |HS〉 and |HT〉 whereand. Bounds on the process fidelitiesFPand average fidelitiesare calculated from the classical fidelities shown under the truth tables. Each truth table requires 16 measurements and each measurement takes 1 s. The count of each high column is around 2,000. Note that for probabilities near zero in the truth tables, we increased the integration time from 1 s to 10 s to improve the statistics. The bases we chose are shown in Figure 4 . The fidelity of these truth tables with the ideal ( F 1 and F 2 ) bound the process fidelity of the gate via: We have also performed full-process tomography on one of these gates (see Methods section). From F P we can calculate the output state fidelity averaged over all input states through the average gate fidelity: where d is the dimension of the gate ( d =4 for a two-qubit gate). The results are shown in Figure 4 . Figure 4: Implementing two-qubit controlled-unitary operations by harnessing entanglement in a larger Hilbert space. ( a–e ) Experimentally measured 'truth tables' for several CU gates. For the inputs of the CH gate | M 〉 and | N 〉 (| J 〉 and | K 〉) are the eigenstates of with +1 and −1 eigenvalues respectively: that is | M 〉=cos( π /8)| H 〉+sin( π /8)| V 〉; | N 〉=sin( π /8)| H 〉−cos( π /8)| V 〉; | J 〉=cos(5 π /8)| H 〉+sin(5 π /8)| V 〉; | K 〉=sin(5 π /8)| H 〉−cos(5 π /8)| V 〉. Note that two different output measurement bases are applied for each truth table of CPhase( π /2) and CPhase( π /4). The red columns correspond to red output labels whereas the blue columns correspond to blue output labels, which include states such as | HL 〉, | HR 〉, | HS 〉 and | HT 〉 where and . Bounds on the process fidelities F P and average fidelities are calculated from the classical fidelities shown under the truth tables. Each truth table requires 16 measurements and each measurement takes 1 s. The count of each high column is around 2,000. Note that for probabilities near zero in the truth tables, we increased the integration time from 1 s to 10 s to improve the statistics. Full size image This method is not limited to realizing CU gates. By changing the values of A 1, A 2, B 1, and B 2, one can implement various two-qubit quantum operations. For example, by setting A 1= A 2=| H 〉〈 H | and B 1= B 2=| V 〉〈 V |, one can realize a very useful quantum gate known as entanglement filter ( EF ) [34] , [35] . An EF is a special (non-unitary) quantum gate which filters multi-qubit states on the basis of correlations. Here our two-photon EF transmits photon pairs, only if they share the same horizontal or vertical polarization, without measuring the polarization state. Compared with the previous method [34] , [35] , our method is simpler and more intuitive. 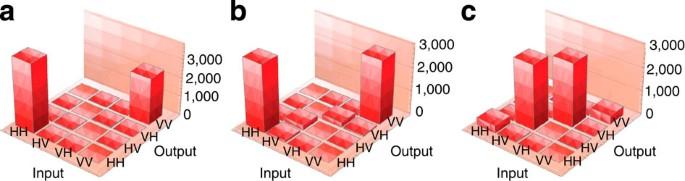Figure 5: An entanglement filter and entanglement splitter. (a) Logical basis truth table for an entanglement filter; the classical fidelity is 98.03±0.17%. (b, c) Logical truth tables for the entanglement splitter. The entanglement splitter's two outputs correspond to two complementary entanglement filters: one transmits |HH〉 and |VV〉 components (b); and the other transmits |HV〉 and |VH〉 components whose truth table is shown in (c); their classical fidelities inH/Vbasis are 90.27±0.37% and 87.38±0.42%, respectively. Here the classical fidelity is defined as the ratio of correctly transmitted photon pairs to the total number of transmitted photon pairs. The data of each column corresponds to 1 s of measurement. We implement this two-photon EF using the setup shown in Figure 3 where A 1= A 2=| H 〉〈 H | and B 1= B 2=| V 〉〈 V | and the results are shown in Figure 5a . Figure 5: An entanglement filter and entanglement splitter. ( a ) Logical basis truth table for an entanglement filter; the classical fidelity is 98.03±0.17%. ( b, c ) Logical truth tables for the entanglement splitter. The entanglement splitter's two outputs correspond to two complementary entanglement filters: one transmits | HH 〉 and | VV 〉 components ( b ); and the other transmits | HV 〉 and | VH 〉 components whose truth table is shown in ( c ); their classical fidelities in H/V basis are 90.27±0.37% and 87.38±0.42%, respectively. Here the classical fidelity is defined as the ratio of correctly transmitted photon pairs to the total number of transmitted photon pairs. The data of each column corresponds to 1 s of measurement. Full size image Another interesting feature of our approach is that the method of realizing a quantum gate is not unique: one can choose different sets of A and B to get the same A+B . Take the two-photon EF, for example. We can realize it in another way by setting A 1= A 2=I and B 1= B 2=Z. This can be verified by comparing the matrix of I I + Z Z with | H 〉〈 H | | H 〉〈 H |+| V 〉〈 V | | V 〉〈 V | that are equivalent up to a constant of order unity. Unlike the first way of realizing an EF, one does not use any projection but only unitary operators, which means that in fact no components are filtered out: Whereas the | H 〉| H 〉 and | V 〉| V 〉 components would exit at 1 and 2 or 1′ and 2′ that corresponds to realizing the quantum gate A+B , the | H 〉| V 〉 and | V 〉| H 〉 components would exit at 1 and 2′ or 1′ and 2 which corresponds to realizing A–B . As the | H 〉| V 〉 and | V 〉| H 〉 components are not filtered out in this case, we call the device an entanglement splitter (ES). The ES operation is deterministic and the experimental data from this gate are shown in Figure 5b and c . Interestingly, the mechanics of the ES can be understood in a different way. The following equations always hold which means ( I I + Z Z )| φ 〉 (or ( I I − Z Z )| φ 〉) is always the eigenstate of operator Z Z with eigenvalue +1 (or −1) no matter what the two-qubit state | φ 〉 is. Then one can deduce that I I + Z Z (or I I − Z Z ) must be a projector that projects any input state to the eigenstate of Z Z with eigenvalue +1 (or −1). As our circuit realizes I I + Z Z and I I − Z Z simultaneously, it can be regarded as an eigenstate generator of, or eigenvalue measuring device for, operator Z Z . One can easily find the above reasoning would hold when replacing Z Z with any two-qubit operator W that fulfill W 2 = I I . This example nicely illustrates the power of linear combination of quantum gates. Although an alternative implementation of an EF has previously been reported [35] (the ES has not been realized), as far as we know, our method is the only solution for constructing these kinds of entangling gates. The imperfections of our experimental results are mainly due to three effects. First, the photons generated in the SPDC source are not completely indistinguishable; second, the phase between the two spatial modes is not perfectly stabilized (to zero); third, the optical components are not perfectly set to the desired values (for example, waveplates' angles). For the EF experiment, A1 , B1 , A2 and B2 are all projectors, and implemented with PBS. In this case, the | H 〉| V 〉 and | V 〉| H 〉 components are nearly completely filtered out and this is not affected by phase errors between the two spatial modes. However in the ES experiment, no component is filtered out, the suppression of | H 〉| V 〉 and | V 〉| H 〉 is all based on interference, which is very sensitive to phase errors between the two spatial modes. The implementation of the CU gates is in between of the two previous cases, where A 1, B 1 are projectors and A 2, B 2 are unitaries. This explains why the fidelity values of the CU gates are higher than those of the ES and lower than those of the EF. Our method will allow simplification of small-scale linear optical circuits. For example, the CNOT gate (or other entangling gates) demonstrated above could be combined with a postselected version of the same gate to perform a sequence of two entangling gates on two photonic qubits. This would require two photons rather than four—which would normally be required for the first gate to be heralded. This type of approach is likely to be of great benefit in circuits of up to 6–10 photons where the appropriate entangled states can be generated [32] and where one can rely on inefficient measurement. This new approach to realizing quantum circuits also enables a quantum state to control the implementation of a quantum gate, thereby opening up the possibility to have truly quantum inputs to quantum information processors. As shown in Figure 2a , if we set the control to be and let the red and blue spatial modes of the target pass through gate O 1 and O 2 instead of I and U respectively, where O 1 and O 2 represent two arbitrary quantum gates, the output state would be , where | ψ 〉 is the initial target state. In some sense, our circuit realizes a peculiar entangled 'state' in which a quantum bit and a quantum gate are entangled (without needing to know what the gate is). This peculiar entanglement connecting a qubit with quantum gates may have some useful implications. An immediate application is to teleport a qubit onto a quantum gate by using this entangled 'state''. In this sense, one can get a quantum gate αO 1 + βO 2 by teleporting a qubit α |0〉+ β |1〉. This is a novel way to control a quantum gate by using a quantum bit that is related to ideas of programmable quantum gate arrays [36] . In summary, we have proposed a different approach to realizing the controlled operations that are at the heart of the majority of important quantum algorithms. With this method, one can directly integrate an arbitrary operation into the circuit to build the corresponding CU gate even if the unitary U is unknown. This is in contrast to other methods that harness extra degrees of freedom [26] , [37] that work only for known single-target qubit unitaries. Our method is not limited to CU gates but can be extended to realize more general entangling gates. We demonstrated the power of this approach by experimentally implementing several high-fidelity two-qubit gates. In each case, the implementation of the control circuit was completely independent of the choice of quantum operation. This method has the potential to change the way we implement quantum circuits for all algorithms and will find a wide range of applications across quantum information science and technology as the complexity of the quantum circuits implemented grows to include more sophisticated algorithms. An alternative experimental demonstration In the experiments described in the main text, we prepared the spatial entangled state as the input ( Fig. 3 ) for implementing the various two-qubit quantum gates, where | φ 〉 is an arbitrary polarization-encoded two-qubit separable state. Here we want to point out that the phase between the two components | φ 〉 1 r ,2 r and | φ 〉 1 b ,2 b was stabilized by using monitoring and feedback method. Although the phase-stabilizing approach is good enough to construct these quantum gates, for application such as the phase estimation algorithm, where phase itself is the target to be measured, a setup with inherent phase stability is required. Here we present an experimental demonstration of the same scheme by using a setup which is inherently phase-stable. Instead of using a type-I SPDC source to produce the spatial entangled photon pairs, we use a type-II SPDC source to get polarization-entangled photon pairs first and then convert them to spatial entangled photons. In this way, we can build a displaced-Sagnac structure in the setup to make the phase stable. 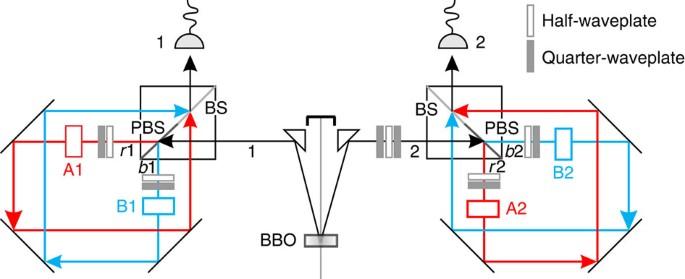Figure 6: Experimental setup in a Sagnac structure. A 60 mW continuous-wave (CW) laser beam with a central wavelength of 404 nm is focused onto a type-II BBO crystal to create entangled photon pairs. The PBS part of the cubes convert the polarization-entangled state to spatial-entangled state. A1, B1, A2 and B2 are four single-qubit gates. By post-selecting the case where the two photons exit at ports 1 and 2, one would effectively realize a two-qubit quantum gate (A1A2+B1B2). The displaced-Sagnac structure makes the phase between modesr1 andb1 (r2 andb2) inherently stable. Figure 6 shows the schematic diagram of our experiment. We use the same continuous wave laser to pump a BBO cystal cut for type-II SPDC and get the two-photon state . Figure 6: Experimental setup in a Sagnac structure. A 60 mW continuous-wave (CW) laser beam with a central wavelength of 404 nm is focused onto a type-II BBO crystal to create entangled photon pairs. The PBS part of the cubes convert the polarization-entangled state to spatial-entangled state. A1, B1, A2 and B2 are four single-qubit gates. By post-selecting the case where the two photons exit at ports 1 and 2, one would effectively realize a two-qubit quantum gate (A1 A2+B1 B2). The displaced-Sagnac structure makes the phase between modes r 1 and b 1 ( r 2 and b 2) inherently stable. Full size image By placing PBS/BS cubes (half-PBS, half-BS) in both arms and by letting the photons pass through the PBS part of the cubes, we get the state . The HWP and quarter-waveplate (QWP) on each path convert the state to that is exactly the same as the spatial entangled state in the original experiments. We let the four spatial modes 1 r , 2 r , 1 b and 2 b pass through four single-qubit gates A 1, A 2, B 1 and B 2, respectively, and then mix the spatial modes 1 r and 2 r (1 b and 2 b ) on the BS part of the cube. By postselecting the case when two photons exit at ports 1 and 2, the quantum operation A+B is obtained. Here we set A 1=| H 〉〈 H |, B 1=| V 〉〈 V |, A 2= I , B 2= X and thus realize a CNOT gate. As the phase θ between r and b modes is inherently stable in this setup, we can now show the variation of the coincidence rates with θ . By setting | φ 〉 to be |+〉| H 〉, the state is obtained. We then place a set of waveplates (QWP, HWP and QWP) in the path of photon 2, as shown, to continuously tune the phase between the spatial modes r and b and measure the |+〉|+〉 and |+〉|−〉 two-photon coincidence rates at the output, where . 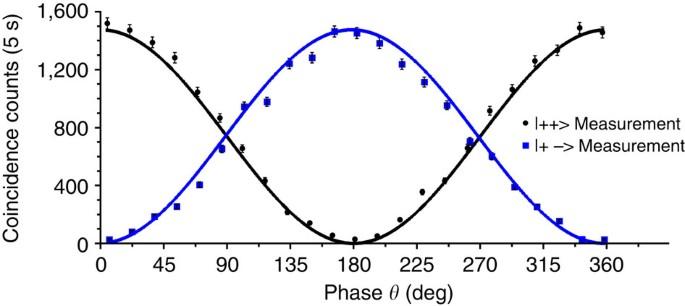Figure 7: Coincidence rates as a function of the phase between spatial modesrandb. The two-photon output state would be, whereθis the relative phase between spatial modesrandb. The coincidence rates of |+〉|+〉 (or |+〉|−〉) would beC(1+cosθ)/2 (orC(1−cosθ)/2) where C is the maximum count rate of |+〉|+〉 (or |+〉|−〉). As shown in Figure 7 , two complementary cosine curves are obtained as expected. Figure 7: Coincidence rates as a function of the phase between spatial modes r and b . The two-photon output state would be , where θ is the relative phase between spatial modes r and b . The coincidence rates of |+〉|+〉 (or |+〉|−〉) would be C (1+cos θ )/2 (or C (1−cos θ )/2) where C is the maximum count rate of |+〉|+〉 (or |+〉|−〉). 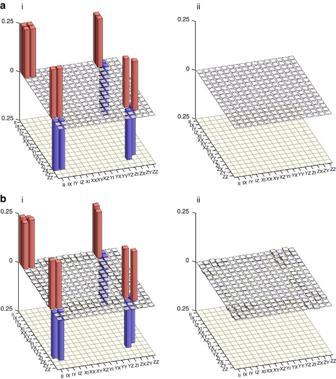Figure 8: Process matrix of the CNOT gate. (a) Ideal process matrix. (b) Maximum-likelihood experimentally reconstructed process matrix. (i) Real and (ii) imaginary parts are shown. We observe a high process fidelity of 96.13±0.17% with the ideal case. The error estimate is obtained by performing many reconstructions with random noise added to the raw data in each case. Matrices are presented in the standard Pauli basis38. Full size image We fully characterize the CNOT gate through quantum process tomography, and the experimentally reconstructed process matrices are shown in Figure 8 . We observe a high process fidelity of 96.13±0.17% with the ideal case. Figure 8: Process matrix of the CNOT gate. ( a ) Ideal process matrix. ( b ) Maximum-likelihood experimentally reconstructed process matrix. (i) Real and (ii) imaginary parts are shown. We observe a high process fidelity of 96.13±0.17% with the ideal case. The error estimate is obtained by performing many reconstructions with random noise added to the raw data in each case. Matrices are presented in the standard Pauli basis [38] . Full size image How to cite this article: Zhou, X.Q. et al . Adding control to arbitrary unknown quantum operations. Nat. Commun. 2:413 doi: 10.1038/ncomms1392 (2011).